Oxidative decomposition mechanisms of lithium carbonate on carbon substrates in lithium battery chemistries Lithium carbonate plays a critical role in both lithium-carbon dioxide and lithium-air batteries as the main discharge product and a product of side reactions, respectively. Understanding the decomposition of lithium carbonate during electrochemical oxidation (during battery charging) is key for improving both chemistries, but the decomposition mechanisms and the role of the carbon substrate remain under debate. Here, we use an in-situ differential electrochemical mass spectrometry-gas chromatography coupling system to quantify the gas evolution during the electrochemical oxidation of lithium carbonate on carbon substrates. Our results show that lithium carbonate decomposes to carbon dioxide and singlet oxygen mainly via an electrochemical process instead of via a chemical process in an electrolyte of lithium bis(trifluoromethanesulfonyl)imide in tetraglyme. Singlet oxygen attacks the carbon substrate and electrolyte to form both carbon dioxide and carbon monoxide—approximately 20% of the net gas evolved originates from these side reactions. Additionally, we show that cobalt(II,III) oxide, a typical oxygen evolution catalyst, stabilizes the precursor of singlet oxygen, thus inhibiting the formation of singlet oxygen and consequent side reactions. Lithium carbonate (Li 2 CO 3 ) is involved in many electrochemical systems, such as lithium-oxygen (Li-O 2 ) batteries [1] , [2] , [3] , [4] , [5] , [6] , [7] , [8] , [9] , [10] , [11] , [12] , [13] , [14] , [15] , lithium-carbon dioxide (Li-CO 2 ) batteries [16] , [17] , [18] , [19] , [20] , [21] , [22] , [23] , [24] , [25] , [26] , [27] , [28] , [29] , [30] , and lithium-ion (Li-ion) batteries [31] , [32] , [33] , [34] , [35] , [36] , [37] , [38] , [39] , [40] , [41] , [42] , [43] . Li 2 CO 3 has extremely low ionic and electronic conductivity due to its wide bandgap [44] , [45] . In Li-O 2 batteries, Li 2 CO 3 mainly results from the side reactions of the reduced oxygen species attacking the electrolytes [1] , [2] , [3] . It not only passivates the electrode surface and polarizes the cell but also consumes the electrolyte, leading to electrolyte depletion and premature cell death. Therefore, Peng et al. referred to Li 2 CO 3 as the “Achilles’ Heel” because it dominates the electrochemical performance of cells [3] . The accumulation of Li 2 CO 3 during cycling has to be well-addressed and resolved in the pursuit of high-performance Li-O 2 batteries. In Li-CO 2 batteries, Li 2 CO 3 is the main desirable discharge product, but the Li 2 CO 3 decomposition during charging has sluggish kinetics and requires a large overpotential. Many efforts have been devoted to designing highly efficient catalysts to reduce the large overpotential [18] , [19] , [20] , [21] , [22] , [23] , [24] , [25] , [26] , [27] , [28] , [29] . In both Li-O 2 batteries and Li-CO 2 batteries, Li 2 CO 3 in the composite electrode needs to be oxidatively decomposed during the charging process, otherwise, it passivates the electrode surface and kills the cells. However, the mechanism of Li 2 CO 3 decomposition is still unclear and this would seriously hinder the research progress. For instance, the role of carbon in the charging process is still under debate. In Li-ion batteries, Li 2 CO 3 is one of the main components of the solid electrolyte interphase of the anode and exists as a surface contaminant present on lithium transition metal oxides used in the cathode thus it influences the cell performance [32] . For instance, the lithium transition metal oxides cathode materials are usually covered with a layer of Li 2 CO 3 due to the residual lithium precursors reacting with CO 2 from the ambient atmosphere [33] , [34] , [35] . Very recently, McCloskey and co-workers have studied the Li 2 CO 3 decomposition mechanism on Li-ion cathodes. Using isotopic labeling, they found that when Li 2 CO 3 is present at the cathode surface, organic fragments containing diatomic oxygen are formed on the cathode surface during the charging process above 4.2 V versus Li + /Li and the diatomic oxygen within these fragments mainly originates from the lithium transition metal oxides lattice and only a minor fraction originates from the Li 2 CO 3 itself [33] , [34] , [35] . In summary, the decomposition of Li 2 CO 3 is so important that it determines the electrochemical performance in many systems. However, its mechanisms are still controversial and not yet well understood, even in the Li-CO 2 cells. Li 2 CO 3 decomposition during the charging process is generally divided into two types, chemical routes, and electrochemical routes [41] , [42] . Recently, Freiberg et al claimed that Li 2 CO 3 decomposition in lithium hexafluorophosphate (LiPF 6 )-ethylene carbonate (EC)-ethylmethyl carbonate (EMC) electrolyte follows a chemical route reacting with H + , which is induced by electrolyte oxidation at >4.6 V [41] . In contrast, Mahne et al. claimed that Li 2 CO 3 decomposition is an electrochemical process [33] , [46] . Here, our results show that the electrolyte salt affects the route and the chemical reaction is likely caused by LiPF 6 , which will be discussed later. So far, several electrochemical mechanisms have been proposed and four possible reaction pathways are summarized below: 
    [ Li_2CO_3-2e^- → 2Li^++CO_2+1/2 O_2                        E_rev=3.8 V ]
 (1) 
    [ Li_2CO_3-2e^-→ 2Li^++CO_2+1/2^1O_2                        E_rev=4.1 V ]
 (1b) 
    [ 2Li_2CO_3+C-4e^-→ 4Li^++3CO_2                   E_rev=2.8 V ]
 (2) 
    2Li_2CO_3-3e^- → 4Li^++2CO_2+O_2^· -
 (3) In Eq. ( 1 a and b), both CO 2 and O 2 formed and it takes 2e – per CO 2 molecule [16] , [17] . The only difference is that O 2 forms as a triplet O 2 in Eq. (1a) and as a singlet O 2 ( 1 O 2 ) in Eq. ( 1b ), respectively. 1 O 2 has been detected at a charging voltage above 3.8 V in the oxidation of Li 2 CO 3 , by using high-performance liquid chromatography (HPLC) and nuclear magnetic resonance spectrometry ( 1 H NMR) analysis [46] . In Eq. ( 2 ), carbon and Li 2 CO 3 were oxidized together to form CO 2 via a 4e – process. That is a common mechanism proposed for the charging process of Li-CO 2 cells. In fact, Eq. ( 2 ) is unlikely to be an elemental reaction, which will be discussed in the text later. In Eq. ( 3 ), oxygen is released in the form of the superoxide radical. Qiao et al. [27] used in situ surface-enhanced Raman spectroscopy to observe the dimethyl sulfone during the charging process and they explained that dimethyl sulfone is attributed to the nucleophilic attack on DMSO solvent from reduced oxygen species (superoxide radicals etc.). Despite the above progress, researchers mainly focus on Li 2 CO 3 and little attention has been paid to the carbon in the charging process. Carbon is always added to the composite electrodes as the conductive additives, however, it is always neglected and its role in Li 2 CO 3 decomposition has not been considered yet. Overall, the mechanism of Li 2 CO 3 decomposition is still under debate and the role of carbon is mysterious. Here, we labeled the Li 2 CO 3 and carbon substrate with 13 C-isotope and qualitatively analyzed the gas products from the decomposition of Li 2 CO 3 , carbon, and electrolyte, respectively. We quantified the gas evolution, particularly CO, during the charging process using an in situ differential electrochemical mass spectroscopy-gas chromatography (DEMS-GC) coupling system. We found that Li 2 CO 3 decomposition is mainly an electrochemical process rather than a chemical process induced by electrolyte oxidation. Li 2 CO 3 decomposes to CO 2 only, but no CO nor O 2 . The oxygen from Li 2 CO 3 is released as highly reactive 1 O 2 , which further attacks the electrolyte and carbon substrate in the composite electrodes to form CO 2 and CO. To study the oxidative decomposition process of Li 2 CO 3 , a cell with a Li 2 CO 3 -carbon composite electrode was constructed and charged. Li 2 CO 3 was electro-oxidized and the gas evolution was quantified. Because both CO and N 2 have the same mass-to-charge ratio of 28 ( m/z = 28), the mass spectrometer typically used in a DEMS system lacks sufficient mass resolution to distinguish the contribution from CO ( m/z = 28.0104) and N 2 ( m/z = 28.0140). Although GC could separate the CO and N 2 , it cannot distinguish and quantify the 13 CO 2 / 13 CO 2 and 12 CO/ 13 CO. Therefore, an in situ DEMS-GC coupling system (Supplementary Fig. 1 ) was used to quantify the evolution of 12 CO, 12 CO 2 , 13 CO, and 13 CO 2 . The details of the experiments are described in Methods. As shown in Supplementary Fig. 2 , after calibration, the CO evolution signals from DEMS and GC experiments are consistent, which provides a reliable amount of CO in the following experiments. Super P carbon (Timcal) was ball milled with Li 2 CO 3 with a mass ratio of 1:1. A Li 2 CO 3 -Super P (1:1) composite electrode was prepared to construct a cell with 1 M lithium bis(trifluoromethane-sulphonyl)imide (LiTFSI)—tetraglyme electrolyte as stated in Methods and the cells were charged by linear sweep voltammetry (LSV). As shown in Fig. 1a , the anodic current for oxidation reaction and gas evolution started at 3.9 V (vs. Li + /Li, all potentials in the text below are versus Li + /Li), which is consistent with the thermodynamic decomposition potential of Li 2 CO 3 (3.82 V according to Eq. 1 ). A control experiment without Li 2 CO 3 was carried out (Supplementary Fig. 3 ). The onset potential of electrolyte decomposition is at 4.3 V. The background current of carbon/electrolyte oxidation at 3.8 V is 10-fold smaller than Li 2 CO 3 decomposition (Fig. 1a ) and there is no CO 2 or O 2 evolution. In Fig. 1a , a large amount of CO 2 and CO were identified as the gas products, which confirms the decomposition of Li 2 CO 3 , consistent with the literature [16] , [17] . According to the mass loading of the electrode (see Methods), ~60% of the preloaded Li 2 CO 3 decomposed eventually. The ratio e-/CO 2 for Fig. 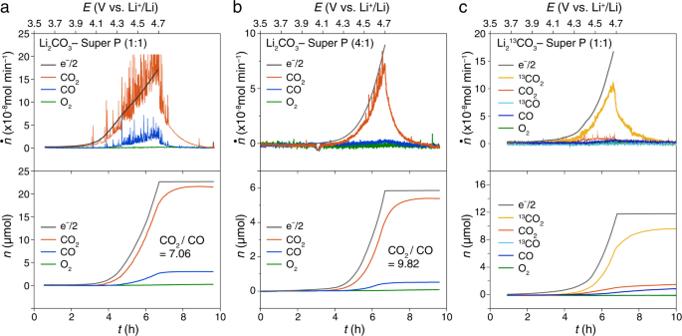Fig. 1: Gas evolution of oxidative decomposition of Li2CO3and Li213CO3. The gas evolution during the charging process of the cells usingaLi2CO3-Super P (1:1),bLi2CO3-Super P (4:1),cLi213CO3-Super P (1:1) composite electrodes in 1 M LiTFSI-tetraglyme. Ar flow rate: 0.5 mL min−1. Sweep rate: 0.05 mV s−1. The molar flux (top panel) of gas evolution was denoted asṅand the charging current is translated toṅelectronand the cumulative mole (bottom panel) of the gas was denoted asn. 1a is 2.1, close to 2e – per CO 2 (Supplementary Table 1 ), suggesting it is an electrochemical process. The deviation is from the electrolyte electro-oxidation without producing CO 2 (Supplementary Fig. 3 ), which is consistent with the literature [41] . The molar flux of both CO 2 (denoted as ṅ CO2 ) and CO (denoted as ṅ CO ) follow the trend of the current during charging (equivalent to ṅ electron ) but they could derive from different processes because of the multisource of the CO 2 and CO evolution. Therefore, we mainly focus on the ratio CO 2 /CO because it helps us to determine the mechanisms (Eqs. 1 – 3 ). The ratio CO 2 /CO exhibits the comparison between Li 2 CO 3 decomposition and other reactions because Li 2 CO 3 decomposition does not form CO, as discussed later. The ratio CO 2 /CO in Fig. 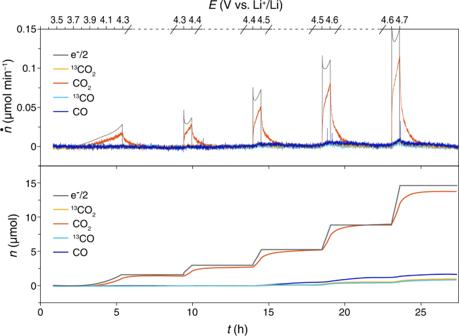Fig. 2: Potential-dependent CO2and CO evolution during the charging process. The gas evolution during the charging process of the cells using Li2CO3-13C (1:1) composite electrode in 1 M LiTFSI-tetraglyme. Sweep rate: 0.05 mV s−1. The cell rested for 4 h after reaching 4.3, 4.4, 4.5, 4.6, and 4.7 V, respectively. Ar flow rate: 0.5 mL min−1. The molar flux (top panel) of gas evolution was denoted asṅand the charging current is translated toṅelectronand the cumulative mole (bottom panel) of the gas was denoted asn. 1a is 7.06 (Supplementary Table 2 ), which does not fit any reaction pathways proposed above. Due to the lack of O 2 evolution, Eq. (1a) could be excluded. The oxygen appears as singlet O 2 ( 1 O 2 ) instead of low-energy triplet O 2 ( 3 O 2 ), which will be discussed in detail later. Fig. 1: Gas evolution of oxidative decomposition of Li 2 CO 3 and Li 2 13 CO 3 . The gas evolution during the charging process of the cells using a Li 2 CO 3 -Super P (1:1), b Li 2 CO 3 -Super P (4:1), c Li 2 13 CO 3 -Super P (1:1) composite electrodes in 1 M LiTFSI-tetraglyme. Ar flow rate: 0.5 mL min −1 . Sweep rate: 0.05 mV s −1 . The molar flux (top panel) of gas evolution was denoted as ṅ and the charging current is translated to ṅ electron and the cumulative mole (bottom panel) of the gas was denoted as n . Full size image To further study the influence of electrode composition on the gas products, the same experiment was conducted using a Li 2 CO 3 -Super P (4:1) composite electrode. As shown in Fig. 1b , similar gas species without O 2 were identified. Because the Li 2 CO 3 -Super P (4:1) composite electrode contains more insulating Li 2 CO 3 solid than that in Li 2 CO 3 -Super P (1:1) electrode, leading to poor solid-solid contact, the charging current and consequent gas evolution in Li 2 CO 3 -Super P (4:1) is one order of magnitude lower than those in Li 2 CO 3 -Super P (1:1) electrode. If the CO 2 and CO came from a certain intermediate or a simple one-step reaction, the same ratio CO 2 /CO would be observed. However, the ratio CO 2 /CO varies with the electrode composition, from 7.06 to 9.82 (Supplementary Table 2 ). This result suggests that the Li 2 CO 3 decomposition is a complicated multistep process, instead of a simple one-step reaction as proposed previously [16] , [17] . Because Li 2 CO 3 , the carbon substrate, and the electrolyte all might contribute to CO 2 and CO evolution, it brings up the confusion about the source of CO 2 and CO, which is the key to addressing the reaction mechanisms. Gas products of Li 2 13 CO 3 decomposition The isotope-labeled Li 2 13 CO 3 was used to identify the decomposition mechanisms of Li 2 CO 3 . The Raman spectrum and XRD pattern of the Li 2 13 CO 3 confirm its composition (Supplementary Fig. 4 ). The 12 C-impurity in Li 2 13 CO 3 is determined by using a mass spectrometer (MS). The details are described in Methods—Isotope impurities. The Li 2 13 CO 3 contains 15% isotope impurity of Li 2 12 CO 3 (Supplementary Fig. 5 ), which would be subtracted from the MS results in the following experiments. Figure 1c exhibits the gas evolution during the charging process of the cell with a Li 2 13 CO 3 -Super P composite electrode. Li 2 13 CO 3 was electro-oxidized and a large amount of 13 CO 2 is identified, which is definitely from the Li 2 13 CO 3 decomposition because both Super P carbon and electrolyte are unlabeled. No O 2 evolution is identified again. 13 CO was not observed as well, indicating that the Li 2 13 CO 3 decomposed to merely 13 CO 2 without 13 CO. The decomposition of Li 2 13 CO 3 (releasing 13 CO 2 ) contributes 79% of the overall CO 2 and CO evolution and it is the dominant process during charging. Meanwhile, some CO 2 and CO from the inevitable decomposition of electrolyte and carbon substrate were identified during charging. 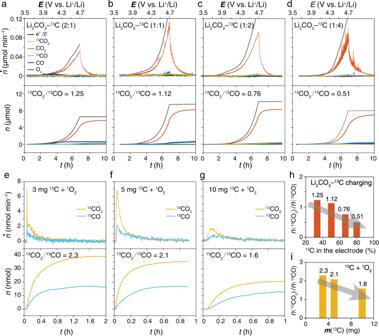Fig. 3: Incomplete oxidation of13C-carbon by singlet O2to form13CO and13CO2. a–dThe gas evolution during the charging process of the cells using the Li2CO3-13C composite electrodes with various mass ratios of Li2CO3/13C,a2:1,b1:1,c1:2,d1:4 in 1 M LiTFSI-tetraglyme.e–g13CO2and13CO evolution of the ex situ chemical reaction between singlet O2and13C-carbon in tetraglyme solution. 22 mg KO2powder was mixed withe3 mg,f5 mg,g10 mg of13C-carbon, respectively, and then 1 mL of LiTFSI-tetraglyme(4 M) was added to react with KO2to form singlet O2. The comparison of ratio13CO2/13CO in (h) ex situ chemical reaction for (e–g) andicharging process for (a–d). The electrolyte/carbon decomposition contributes to approximately one-fifth of total gas evolution (Supplementary Table 3 ), which is a high ratio of side reactions. 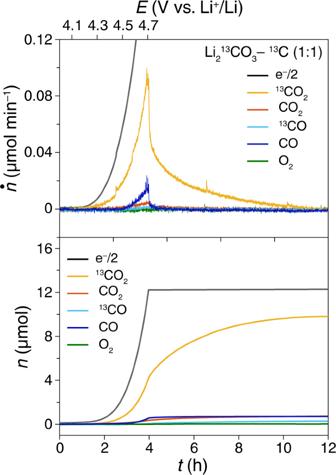Fig. 4: The gas evolution of the electrolyte decomposition. The gas evolution during the charging process of the cells using Li213CO3-13C-carbon (1:1) composite electrode in 1 M LiTFSI-tetraglyme. Ar flow rate: 0.5 mL min−1. Sweep rate: 0.05 mV s−1. The molar flux (top panel) of gas evolution was denoted asṅand the charging current is translated toṅelectronand the cumulative mole (bottom panel) of the gas was denoted asn. The unlabeled CO2and CO are contributed by electrolyte decomposition. In the Li-CO 2 chemistry with lithium carbonate isotopically labeled with 13 C on an unlabeled carbon substrate (which we write here as 12 C for simplicity), Li 2 13 CO 3 is posited to decompose together with the carbon substrate in the following reaction: 
    2Li_2 ^13CO_3+ ^12C-4e^-→ 4Li^++2 ^13CO_2+ ^12CO_2
 (4) If it was the case, the ratio between 13 CO 2 and 12 CO 2 is expected to be about 2/1, but we find a ratio of 6.1/1 (Supplementary Table 4 ), much higher than 2/1 because 12 C does not transform to sufficient 12 CO 2 . This result suggests that the decomposition of the Li 2 CO 3 -C electrode is a complicated reaction instead of a simple reaction with known stoichiometric numbers like Eq. ( 4 ). Therefore, the contribution of the C substrate during the charging process is the key to demystifying the reaction mechanisms. Decomposition of 13 C-carbon substrate To determine the contribution of carbon in this reaction, the same experiments were carried out again but by replacing the Super P carbon substrate with 13 C-carbon and leaving the lithium carbonate and electrolyte unlabeled. The 13 C-carbon contains 1.5% of 12 C impurity as shown in Supplementary Fig. 6 . As shown in Fig. 2 and Supplementary Fig. 7 , both 13 CO 2 and 13 CO evolved during the charging process and the rest of CO 2 and CO evolution came from the decomposition of Li 2 CO 3 and electrolyte. As the only source of 13 C-isotope, 13 C is oxidized to release both 13 CO 2 and 13 CO during the charging process. The formation of 13 CO exhibits that the 13 C is oxidized incompletely like an incomplete combustion reaction. The 13 C substrate could be oxidized either electrochemically by potential or chemically by oxidative agents that are formed in the previous steps. If 13 C is oxidized electrochemically, the ratio 13 CO 2 / 13 CO would depend on the potential (Fig. 2 ). If 13 C is oxidized chemically by oxidative agents like 1 O 2 and superoxide species, which are generated during the charging process, the electrode composition affects the ratio between 13 CO 2 and 13 CO. Fig. 2: Potential-dependent CO 2 and CO evolution during the charging process. The gas evolution during the charging process of the cells using Li 2 CO 3 - 13 C (1:1) composite electrode in 1 M LiTFSI-tetraglyme. Sweep rate: 0.05 mV s −1 . The cell rested for 4 h after reaching 4.3, 4.4, 4.5, 4.6, and 4.7 V, respectively. Ar flow rate: 0.5 mL min −1 . The molar flux (top panel) of gas evolution was denoted as ṅ and the charging current is translated to ṅ electron and the cumulative mole (bottom panel) of the gas was denoted as n . Full size image Impact of the potential on the decomposition of 13 C-carbon substrate Due to the high equilibrium potential of Li 2 CO 3 decomposition (3.82 V), the cell potential could affect the decomposition reactions and thus affect the formation of 13 CO 2 and 13 CO at different potentials during the charging process. Therefore, a cell with Li 2 CO 3 - Super P composite electrode was charged with LSV from 4.3 to 4.7 V and the gas evolution was measured. The cell was rested for 4 h after reaching 4.3, 4.4, 4.5, 4.6, and 4.7 V, respectively, to obtain a low background of gas evolution. The cumulative molar of gas evolution at various potential stages is shown in Fig. 2 . The amount of CO 2 from Li 2 CO 3 decomposition increased when the potential increased. The higher the potential was, the more CO 2 evolved, in accord with the accelerating decomposition of Li 2 CO 3 . Meanwhile, 13 CO 2 and 13 CO evolved simultaneously and their amount increased together with the CO 2 evolution when the potential increased. Supplementary Fig. 7 shows the gas evolution at various stages of the charging process from 4.4 to 4.7 V. The amount of 13 CO 2 and 13 CO evolution increased with the rising potential up to 4.7 V. This increase is probably because more singlet oxygen forms at a higher potential, which leads to more severe carbon and electrolyte degradation. Although both 13 CO 2 and 13 CO increased, the ratio 13 CO 2 / 13 CO remains almost identical at these stages. This result suggests that the 13 CO 2 and 13 CO likely originated from the same chemical reaction. To check whether 13 C is oxidized to any solid byproducts, the cell was dissembled at the end of charging and the composite electrode was collected to further quantify the remained solid by-product of inorganic/organic carbon as described in Methods—Quantification of the solid byproducts. Neither Li 2 13 CO 3 (Supplementary Fig. 8a ) nor organic 13 C-carbonates (Supplementary Fig. 8b ) were detected in the charged electrode, indicating that the 13 C did not oxidize to any solid by-products, i.e., inorganic and organic carbonates. Only unlabeled inorganic Li 2 CO 3 and organic carbonate were identified, which are from undecomposed Li 2 CO 3 and electrolyte decomposition. The incomplete decomposition of Li 2 CO 3 may be due to the poor solid-solid contact between the carbon substrate and Li 2 CO 3 during the charging process. It is unlikely to decompose all Li 2 CO 3 even up to 4.7 V, which is consistent with the literature [41] . Therefore, as only 13 CO and 13 CO 2 and no 13 C-containing solid products are detected when using 13 C as the carbon substrate, the carbon substrate is only oxidized to gaseous carbon monoxide and carbon dioxide during charge in the presence of lithium carbonate and the 1 M LiTFSI-tetraglyme electrolyte. Previous results showed that the functional groups at the carbon surface dominated the decomposition of the carbon substrate [47] . Therefore, the Raman and XPS spectra of 13 C and Super P are recorded to show their surface condition (Supplementary Fig. 9 ). D-band and G-band of 13 C were observed at 1289 and 1507 cm –1 , respectively, in the Raman spectrum (Supplementary Fig. 9a ). Both D-band and G-band drift in the negative direction due to the isotope effect. The intensity of the D-band and G-band ( I D /I G ) typically represents the disorderliness and amounts of defects in the carbon structure. Here, 13 C and Super P carbon show the same I D /I G of 1.20, which indicates the same degree of disorderliness and a similar amount of defects from the surface of 13 C and Super P. Similar XPS spectra are shown in Supplementary Fig. 9b , confirming the similar surface groups of these two carbon substrates. Therefore, 3 C and Super P have similar surface functional groups and they are likely to exhibit similar behavior in this carbon decomposition on charge. Impact of the ratio of Li 2 CO 3 and carbon on the gas evolution Although the 13 C carbon substrate oxidized to 13 CO and 13 CO 2 , its decomposition pathway is still ambiguous. It might be a pathway similar to the incomplete combustion reaction. Alternatively, 13 CO and 13 CO 2 might be derived from a reaction intermediate with known structures like oxalate (C 2 O 4 2− ). To clarify the pathway, we studied the gas products of four Li 2 CO 3 - 13 C composite electrodes with various mass ratios of Li 2 CO 3 / 13 C from 2:1 to 1:4 (Fig. 3 ). Overall, the carbon decomposition contributes to about 10% of the total gas evolution and the exact contribution depends on the composition of the electrodes (Supplementary Table 3 ). When the composite electrode contains less Li 2 CO 3 , ratio 13 CO 2 / 13 CO decreases from 1.25 to 0.51 (Fig. 3h ), indicating the extent of oxidation of 13 C is restricted by the amount of Li 2 CO 3 in the composite electrodes. Otherwise, the 13 C would be completely oxidized to 13 CO 2 instead of the mixture of 13 CO 2 and 13 CO. This varying ratio 13 CO 2 / 13 CO confirms that the overall reaction is a multistep reaction, rather than forming a complex intermediate like C 2 O 4 2− which should give a certain ratio 13 CO 2 / 13 CO independent of the ratio of Li 2 CO 3 / 13 C. The 13 C is highly likely to be oxidized by the oxidative intermediates from Li 2 CO 3 decomposition. Therefore, as ratio 13 CO 2 / 13 CO varied with varying composition of the Li 2 CO 3 - 13 C composite electrode, we argue that the amount of Li 2 CO 3 present in the electrode, and thus the amount of oxidative intermediates from Li 2 CO 3 decomposition, influences the decomposition route of the carbon substrate. Fig. 3: Incomplete oxidation of 13 C-carbon by singlet O 2 to form 13 CO and 13 CO 2 . a – d The gas evolution during the charging process of the cells using the Li 2 CO 3 - 13 C composite electrodes with various mass ratios of Li 2 CO 3 / 13 C, a 2:1, b 1:1, c 1:2, d 1:4 in 1 M LiTFSI-tetraglyme. e – g 13 CO 2 and 13 CO evolution of the ex situ chemical reaction between singlet O 2 and 13 C-carbon in tetraglyme solution. 22 mg KO 2 powder was mixed with e 3 mg, f 5 mg, g 10 mg of 13 C-carbon, respectively, and then 1 mL of LiTFSI-tetraglyme(4 M) was added to react with KO 2 to form singlet O 2 . The comparison of ratio 13 CO 2 / 13 CO in ( h ) ex situ chemical reaction for ( e – g ) and i charging process for ( a – d ). Full size image Oxidation of 13 C-carbon by 1 O 2 and superoxide Both 1 O 2 and superoxide are reactive intermediates formed during the discharge and charging process in Li-air batteries, which could result in the decomposition of the carbon substrate [48] , [49] , [50] , [51] , [52] . 1 O 2 could attack the electrolytes and the electrodes as a strong oxidative species. Here, 9,10-dimethylanthracene (DMA), a molecular trap for 1 O 2 , is used to identify the 1 O 2 during electrochemical oxidation for the Li 2 CO 3 -C composite electrodes (see Methods—Identification of 1 O 2 ). When 1 O 2 forms, it rapidly reacts with DMA to form DMAO 2 , which could be identified in the 1 H NMR spectrum. Here, at the end of the charging process, the electrolyte with DMA in the cell was extracted and its 1 H NMR spectrum (Supplementary Fig. 10 ) shows that DMAO 2 has formed, which confirms the formation of 1 O 2 during the charging process. Once 1 O 2 forms, 1 O 2 attacks carbon and releases 13 CO and 13 CO 2 . Here, to study the contribution of 1 O 2 and KO 2 to carbon decomposition, 1 O 2 and KO 2 were respectively used to react with 13 C as ex situ chemical experiments. 1 O 2 is produced from the disproportionation of superoxide species [47] (The reaction between KO 2 and Li + in this work). More details are described in Methods—Chemical experiments between reactive oxygen species and carbon. The gas evolutions of 13 CO 2 , 13 CO, 12 CO 2 , and O 2 in the reaction between 1 O 2 and 13 C are shown in Fig. 3e–g and Supplementary Fig. 11 . Figure 3e–g show both 13 CO and 13 CO 2 evolution, which confirms the incomplete oxidation of 13 C-carbon by 1 O 2 . The formation efficiency of 1 O 2 by disproportionation in solution is low, therefore, most O 2 is released as 3 O 2 (Supplementary Fig. 11 ). Because 1 O 2 is formed in the electrolyte solution rather than at the surface of 13 C, fresh 1 O 2 is more likely to attack the electrolyte than the 13 C, forming a large amount of CO 2 . In addition, because a large amount of carbon makes the suspension viscous, the total amount of 13 CO and 13 CO 2 slightly decreased with the increase of 13 C. When the amount of 13 C increased, more 13 CO formed and the ratio 13 CO 2 / 13 CO decreased (Fig. 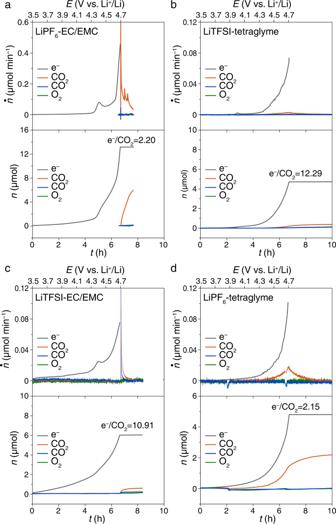Fig. 5: Impact of electrolyte salts and solvents on the gas evolution of chemical decomposition of Li2CO3. The gas evolution during the charging process of the cells using Super P-PTFE composite electrodes without direct contact of Li2CO3ina1 M LiPF6-EC/EMC,b1 M LiTFSI-tetraglyme.c1 M LiTFSI-EC/EMC, andd1 M LiPF6-tetraglyme. 20 mg of commercial Li2CO3was separated from the Super P-PTFE electrode with a Celgard separator to allow a chemical decomposition but not electro-oxidation decomposition. Ar flow rate: 0.5 mL min−1. Sweep rate: 0.05 mV s−1. The molar flux (top panel) of gas evolution was denoted asṅand the charging current is translated toṅelectronand the cumulative mole (bottom panel) of the gas was denoted asn. 3i and Supplementary Table 5 ). Both the in situ electrochemical charging experiments (Fig. 3h ) and ex situ chemical experiments (Fig. 3i ) show the same decreasing trend of ratio 13 CO 2 / 13 CO with the increase of the amount of 13 C relative to 1 O 2 or Li 2 CO 3 . On the other hand, to further exclude the contribution from superoxide species, the same chemical experiments were carried out but replaced 1 O 2 with O 2 – (sol) . KO 2 was dissolved in tetraglyme and crown ether was added to maximize the concentration of the O 2 − (sol) in the solution. As shown in Supplementary Fig. 12 , only 13 CO but no 13 CO 2 was identified, which suggests that O 2 − (sol) is incapable to oxidize 13 C to 13 CO 2 . In summary, the detected 13 CO and 13 CO 2 come from the side-reaction of 1 O 2 attacking the 13 C substrate (Eq. 6 ). Herein, we simulate the chemical reaction between 1 O 2 and 13 C without applying potential, however, the potential applied in the charging process could make the real side-reaction more complicated. More 1 O 2 might be produced at a higher potential. It is noted that oxygenated byproducts from chemical reactions with 1 O 2 could first be produced and then electro-oxidatively decomposed [48] , [49] . The CO and CO 2 evolution of electrolyte decomposition The electrolyte decomposition during the oxidation of Li 2 CO 3 on charge is inevitable and should not be ignored. A cell with Li 2 13 CO 3 - 13 C composite electrode was charged to quantify the contribution from electrolyte degradation (Fig. 4 ). Because the entire composite electrode is labeled with 13 C isotope, the 12 CO 2 must come from the decomposition of the tetraglyme electrolyte. 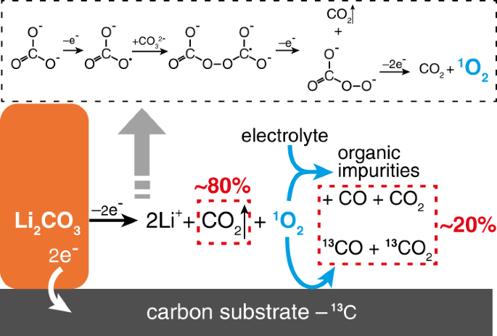Fig. 6: Schematics of the Li2CO3decomposition on the charging process. Li2CO3is electro-oxidized to form CO2and singlet O2(1O2). A possible pathway is proposed in the dash line box.1O2is highly reactive and it attacks the electrolyte and the carbon substrate to form carbon monoxide and carbon dioxide, which contribute to ~20% of the overall gas evolution. Figure 4 shows that 12 CO 2 and 12 CO from the electrolyte decomposition contribute ~12% to the total gas evolution (Supplementary Table 6 ). The ratio between carbon dioxide species ( 12 CO 2 + 13 CO 2 ) and carbon monoxide species ( 12 CO + 13 CO) is 7.76, which is in accord with the ratio CO 2 /CO of 7.06 in the Li 2 CO 3 - Super P (1:1) composite electrode, as stated in Supplementary Table 2 . Fig. 4: The gas evolution of the electrolyte decomposition. The gas evolution during the charging process of the cells using Li 2 13 CO 3 - 13 C-carbon (1:1) composite electrode in 1 M LiTFSI-tetraglyme. Ar flow rate: 0.5 mL min −1 . Sweep rate: 0.05 mV s −1 . The molar flux (top panel) of gas evolution was denoted as ṅ and the charging current is translated to ṅ electron and the cumulative mole (bottom panel) of the gas was denoted as n . The unlabeled CO 2 and CO are contributed by electrolyte decomposition. Full size image As discussed above, the decomposition of Li 2 CO 3 and carbon substrate contributes to 79% and ~10%, respectively, of the total gas evolution. The side-reactions of carbon depend on the electrode composition because this charging process highly depends on the solid-solid contact between Li 2 CO 3 and carbon substrate. The exact ratios of decomposition of individual components were not completely identical in each experiment because the nature of Li 2 CO 3 decomposition is based on the solid-solid contact. At some contacting points, the charging process will stop due to the large overpotential caused by the restricted solid-solid contact. The sum of gas evolution from Li 2 CO 3 , carbon, and electrolyte is ~100%, which confirms the reliability of individual measurements. Although an important consideration, full understanding of electrolyte decomposition is not our focus in this work. Therefore, to ensure that it does not affect the major gas evolution from Li 2 CO 3 and C, we quantified the gas by-products and solid by-products from the electrolyte decomposition without further analyzing the liquid by-products dissolved in the solvent. The solid by-products, like Li 2 CO 3 and organic carbon residuals in the composite electrode at the end of the charge, were quantified respectively. As shown in Supplementary Fig. 13 , approximately one-third of Li 2 13 CO 3 is unreacted and remained in the electrode and a trace amount (<0.1 μmol) of organic carbonate were identified. This result indicates that there is no exchange of 12 C/ 13 C between the electrolyte and Li 2 CO 3 /C. Electrochemical vs. chemical pathways of Li 2 CO 3 decomposition Here our results show that Li 2 CO 3 decomposition in the ether-based electrolyte is mainly an electrochemical process, which is in good agreement with Kaufman et al. [33] , but Freiberg et al claimed that Li 2 CO 3 decomposition was a chemical process in LiPF 6 carbonate-based electrolyte and it was induced by water [41] . They argued that the electrolyte was oxidized and decomposed on high potential and it formed some proton-derivatives which chemically react with Li 2 CO 3 to evolve CO 2 . To study the reasons of these contradicting results, we conducted a series of comparative experiments. Firstly, to avoid the direct participation of water in Li 2 CO 3 decomposition, we carried out a chemical reaction between the commercial Li 2 CO 3 and 1 M LiTFSI tetraglyme electrolyte with 1000 ppm and 5000 ppm H 2 O, respectively, and the gas evolution was recorded. The result in Supplementary Fig. 14 indicates that no CO 2 and O 2 were detected even if there were lots of protons (from water) in the electrolyte. Then, to check the impact of potential, a cell with blank carbon (Super P or 13 C) electrode without Li 2 CO 3 but with 1000 ppm of H 2 O in the electrolyte and the gas evolution was recorded, Supplementary Fig. 15 . No O 2 and CO 2 evolved during the charging process below 4.7 V. Interestingly, in the presence of 1000 ppm H 2 O, the onset potentials of electrolyte decomposition drifted to a lower potential of 3.8 V, compared with 4.1 V without H 2 O. This result implies that H 2 O encourages the electro-oxidation of the electrolyte but there is still no gas evolution below 4.5 V. Learning from Freiberg’s work, we decomposed Li 2 CO 3 without direct electric contact to confirm the chemical mechanism [41] . Briefly, an extra Celgrad membrane was placed between Li 2 CO 3 powder and the blank carbon composite electrode to separate them. On one hand, the Li 2 CO 3 cannot be electro-oxidized due to the lack of direct electronic contact with the carbon electrode. On the other hand, the porous Celgard membrane allows the electrolyte decomposition byproducts that form at the carbon composite electrode to diffuse across the Celgard and react with Li 2 CO 3 . For comparison, in the LiPF 6 -ethylene carbonate (EC)/ethyl methyl carbonate (DMC) electrolyte, the same setup was used but the gas evolution was analyzed at the end of the charging process due to the volatility of the EMC. Because the Li 2 CO 3 is separated from the carbon electrode, it cannot be electro-oxidized. However, a large amount of CO 2 evolution was identified (Fig. 5a ) above 4.3 V, suggesting the chemical decomposition of Li 2 CO 3 by the electrolyte decomposition byproducts at high potential. This result is consistent with Freiberg’s work [41] . The ratio e − /CO 2 is 2.20, in good agreement with the literature [41] but it does not mean that Li 2 CO 3 is electro-oxidized via a 2-e process. Instead, the electrolyte decomposition is likely to produce active H + at a ratio e − /H+ of 1 and the H + reacts with Li 2 CO 3 to release CO 2 at a ratio H+/CO 2 of 2 [41] . Therefore, here the ratio e − /CO 2 is just used for comparison between these four cells. Here, the chemical pathway does not take place until a high potential over 4.3 V when the electrolyte was electro-oxidized first. For comparison, the CO 2 evolution in the charging process starts from ~3.9 V (Figs. 1 – 3 ), which is too low to electro-oxidize the electrolyte. Therefore, the Li 2 CO 3 decomposition at low potential <3.9 V is dominated by the electrochemical pathway, instead of by a chemical pathway induced by electrolyte degradation by-products. Fig. 5: Impact of electrolyte salts and solvents on the gas evolution of chemical decomposition of Li 2 CO 3 . The gas evolution during the charging process of the cells using Super P-PTFE composite electrodes without direct contact of Li 2 CO 3 in a 1 M LiPF 6 -EC/EMC, b 1 M LiTFSI-tetraglyme. c 1 M LiTFSI-EC/EMC, and d 1 M LiPF 6 -tetraglyme. 20 mg of commercial Li 2 CO 3 was separated from the Super P-PTFE electrode with a Celgard separator to allow a chemical decomposition but not electro-oxidation decomposition. Ar flow rate: 0.5 mL min −1 . Sweep rate: 0.05 mV s −1 . The molar flux (top panel) of gas evolution was denoted as ṅ and the charging current is translated to ṅ electron and the cumulative mole (bottom panel) of the gas was denoted as n . Full size image On the contrary, the same experiment but with LiTFSI-tetraglyme electrolyte shows little CO 2 evolution (Fig. 5b ), which makes a sharp comparison to the LiPF 6 -EC/EMC electrolyte. In LiTFSI-tetraglyme electrolyte. CO 2 evolved from 4.3 V, indicating the decomposition of electrolytes at high potential could induce the chemical decomposition of Li 2 CO 3 . However, the ratio e − /CO 2 is 12.29, much higher than that in LiPF 6 -EC/EMC. In addition, the total amount of CO 2 is as low as 0.4 μmol, <2% of the CO 2 evolution in the Super P-Li 2 CO 3 electrode, Fig. 1a . This distinct comparison indicates that the reaction mechanisms of Li 2 CO 3 decomposition are completely different in LiPF 6 -EC/EMC and LiTFSI-tetraglyme electrolytes. The chemical pathway proposed by Freiberg is not applicable for tetraglyme-based electrolytes. The difference is due to either the Li salts or the solvents. To find out whether the Li salts or the solvents make the difference, the salts were exchanged in these electrolytes and LiTFSI-EC/EMC and LiFP 6 -tetraglyme were used, Fig. 5c and d . Interestingly, the LiPF 6 -tetraglyme shows much CO 2 evolution similar to LiPF 6 -EC/EMC. Meanwhile, LiTFSI-EC/EMC shows little CO 2 evolution similar to LiTFSI-tetraglyme. The cells using LiPF 6 salt show a large amount of CO 2 evolution. The electrolytes used in this work were all dried and the water concentrations were below 4 ppm (Karl-Fischer titration). Therefore, this chemical mechanism could be due to the LiPF 6 salt itself or its impurities because LiPF 6 is difficult to purify [53] . Freiberg et al. also proposed that the chemical pathway involving LiPF 6 salt [41] . In the rest of this work, we used LiTFSI in tetraglyme as the electrolyte, thus excluding any possible effects of LiPF 6 on our results. As little CO 2 was evolved in the Celgard-separated experiment with LiTFSI-based electrolytes, our results provide evidence that Li 2 CO 3 decomposition in LiTFSI-tetraglyme electrolytes is dominated by an electrochemical rather than chemical process. We propose the following reactions for the electrochemical decomposition of Li 2 CO 3 on carbon substrates: 
    Li_2CO_3-2e^-→CO_2+2Li^++1/2 ^1O_2
 (5) 
    (1-x/2) ^1O_2+C→ (1-x)CO_2+x CO
 (6) 
    ^1O_2+electrolyte→CO_2+CO+byproducts
 (7) Li 2 CO 3 is oxidized at high potentials to form CO 2 and aggressive 1 O 2 (Eq. 5 ), Fig. 6 . 1 O 2 attacks carbon substrate (Eq. 6 ) and electrolyte (Eq. 7 ) simultaneously like incomplete combustion reactions, leading to further side reactions forming CO 2 and CO. It should be noted here, Eq. ( 7 ) is just a schematics equation instead of a proper stoichiometric equation for an elementary reaction because we do not completely know all byproducts from electrolyte decomposition. The exact ratio CO 2 /CO depends on the ratio between formed 1 O 2 , the carbon substrate/electrolyte, namely the electrode composition, but not on the cell potentials. Although the carbon substrate is eventually oxidized to CO 2 and CO, the carbon does not directly participate in the electro-oxidation of Li 2 CO 3 as has been proposed in the literature [28] . As we mentioned above, the Eq. ( 2 ) could be recognized as a combination of Eq. ( 5 ) and Eq. ( 6 ) when x is equal to zero in Eq. ( 6 ). In this case, the reactive intermediate 1 O 2 reacts with carbon to produce only CO 2 instead of a mixture of CO 2 and CO. However, our chemical reaction between 1 O 2 and 13 C shows both 13 CO 2 and 13 CO evolution (Supplementary Fig. 11 ). If a highly reactive intermediate other than 1 O 2 forms in the Li 2 CO 3 decomposition and rapidly attacks carbon to just CO 2 , Eq. ( 2 ) could establish and contribute to a parallel pathway with Eq. ( 1 ) in Li 2 CO 3 decomposition. However, there is so far no evidence of such a highly reactive intermediate. Fig. 6: Schematics of the Li 2 CO 3 decomposition on the charging process. Li 2 CO 3 is electro-oxidized to form CO 2 and singlet O 2 ( 1 O 2 ). A possible pathway is proposed in the dash line box. 1 O 2 is highly reactive and it attacks the electrolyte and the carbon substrate to form carbon monoxide and carbon dioxide, which contribute to ~20% of the overall gas evolution. Full size image Overall, during the charging process of the cell with a Li 2 CO 3 -carbon composite electrode in LiTFSI-tetraglyme electrolyte, Li 2 CO 3 decomposition contributes the major CO 2 evolution (~80%), and the carbon substrate and electrolyte decomposition share the rest ~20% of gas evolution. Therefore, in the charging process of Li-air batteries and Li-CO 2 batteries, the decomposition of carbon substrate and the electrolyte is inevitable and contributes to a significant amount of CO 2 and CO unless the 1 O 2 can be suppressed. Implications for batteries Although Li 2 CO 3 can be decomposed during the charging process, it is accompanied by severe side reactions by 1 O 2 (~20% of the total gas evolution) and leads to deterioration of cell performance. Here, we focus on Li-air and Li-CO 2 batteries. In Li-air batteries, Li 2 CO 3 is a major by-product and it passivates the electrode surface and kills the cells, which brings us to a dilemma. On one hand, if Li 2 CO 3 is not decomposed during the charging process, Li 2 CO 3 will rapidly accumulate during cell cycling and thus completely passivate the electrode. On the other hand, if Li 2 CO 3 is decomposed during the charging process, it results in more side-reactions and thus accelerates cell deterioration. This effect is more significant in Li-CO 2 batteries because Li 2 CO 3 and carbon form are supposed to be the main discharge products. Therefore, a reversible decomposition of Li 2 CO 3 and carbon is desired in the following charging process [16] , [17] . However, during the charging process, the discharge reaction cannot be completely reversed because the carbon does not directly participate in the Li 2 CO 3 decomposition reactions. The carbon substrate is oxidized by the 1 O 2 intermediate to CO 2 and CO. Meanwhile, the aggressive 1 O 2 attacks the electrolyte, leading to the depletion of the electrolyte and consequently cell failure. If the electrolytes and salts in the cells are sufficiently stable, e.g., solid-state electrolyte, the molten-salt electrolyte of LiNO 3 -KNO 3 , etc, the side-reactions with electrolyte could be avoided and 1 O 2 quenches to 3 O 2 . Recently, Zhang’s group observed the O 2 evolution when charging Li 2 CO 3 in the cell using a solid-state electrolyte [54] . Due to the stability of inorganic solid-state electrolyte, 1 O 2 had nothing to attack and eventually was quenched to 3 O 2 . However, even in this case, the 1 O 2 would oxidize the carbon substrate and thus the cell deterioration cannot be completely inhibited. Therefore, the key to pursuing a better charging process is to design a catalyst that suppresses the formation of 1 O 2 rather than simply facilitates the kinetics of Li 2 CO 3 decomposition and thus decreases the overpotentials. For instance, some redox mediators (RM) with moderate O 2 binding energy could be applied to inhibit forming 1 O 2 and encourage 3 O 2 evolution by replacing the 1 O 2 precursor (e.g. CO 4 2− ) with a low-energy RM-involved intermediate, just like the way 2,5-di-tert-butyl-1,4-benzoquinone does to O 2 − [55] . Alternatively, some solid catalysts with suitable O 2 binding energy could bind 1 O 2 precursor (the key reaction intermediator of Li 2 CO 3 decomposition) in order to lower the energy and stabilize the precursor before it transforms to 1 O 2 . The ratio of 1 O 2 in the final product will decrease when the energy of the 1 O 2 precursor decreases. Very recently, Hu’s group used operando electron paramagnetic resonance to show that Co 3 O 4 inhibited the 1 O 2 formation during the charging process of Li-O 2 cells [56] . Here, we added some Co 3 O 4 nanoparticles to the Li 2 CO 3 -Super P composite electrode and then charged the electrode. As shown in Supplementary Fig. 16a , some O 2 was identified during the charging process. While the control experiment of charging the Co 3 O 4 electrode itself without Li 2 CO 3 exhibits no O 2 evolution, Supplementary Fig. 16b . This result confirms that the Co 3 O 4 catalyst successfully interacts with the precursor of forming 1 O 2 during the Li 2 CO 3 decomposition and thus suppresses 1 O 2 formation. On the other hand, the CO evolution with Co 3 O 4 is only half of that without Co 3 O 4 , whereas similar CO 2 evolutions were identified in both experiments. Because CO is from side-reactions of 1 O 2 attacks electrolyte/carbon substrate, decreased CO evolution confirms that 1 O 2 formation was partially inhibited and thus fewer side-reactions of 1 O 2 attacking the carbon substrate and the electrolyte were detected than the counterpart without Co 3 O 4 , Supplementary Fig. 17 . Our results are in good agreement with Hu’s group results [55] . Although the 1 O 2 formation and CO evolution cannot be completely inhibited, the Co 3 O 4 does make some effects by stabilizing the reaction intermediates of forming 1 O 2 and thus encouraging the evolution of 3 O 2 . This example confirms the feasibility of this strategy to promote the Li 2 CO 3 decomposition with less parasitic 1 O 2 , however further studies are needed to look for more effective catalysts to avoid the side-reaction caused by 1 O 2 . To explore the decomposition mechanisms of the Li 2 CO 3 and clarify the role of carbon substrate in the charging process of Li 2 CO 3 -carbon composite electrodes in LiTFSI-tetraglyme electrolyte, we did a set of in situ DEM-GC experiments with the 13 C isotope-labeled composite electrodes to systematically isolate each component of the cell. The gas evolution during the charging process, including CO, CO 2 , 13 CO, 13 CO 2 , and O 2 was quantified. Li 2 CO 3 decomposed to release CO 2 at an onset potential of 3.8 V mainly via an electrochemical mechanism. The chemical mechanism of Li 2 CO 3 decomposition in literature could take place in the presence of LiPF 6 due to LiPF 6 itself or its impurities. Carbon substrate did not directly participate in the decomposition of Li 2 CO 3 , that is to say, carbon did not react with Li 2 CO 3 in a single step to form CO 2 as desired. On the contrary, this process is a multistep reaction. In the first step, Li 2 CO 3 was oxidized to CO 2 and 1 O 2 . Then, the 1 O 2 simultaneously oxidized the carbon substrate and electrolyte to form CO 2 and CO as gaseous side products. Approximately 80% of the net/cumulative CO 2 evolution is contributed by the Li 2 CO 3 decomposition and the rest ~20% is contributed by the decomposition of the carbon substrate and the electrolyte, which cannot be ignored in batteries, particularly in Li-CO 2 batteries. In this work, we clarify the reaction mechanisms of the Li 2 CO 3 decomposition during the charging process and exhibit the role of carbon in this process. This finding establishes a detailed picture of the decomposition pathways of Li 2 CO 3 which enables strategy for the design of highly efficient cathode catalysts for Li-air and Li-CO 2 batteries. Materials Lithium carbonate (Li 2 CO 3 ), potassium superoxide (KO 2 ), lithium bis(trifluoromethane)sulfonamide (LiTFSI), 9,10-dimethylanthracene (DMA), and Co 3 O 4 were purchased from Sigma-Aldrich. Li 2 13 CO 3 and 13 C were purchased from the Cambridge Isotope Ltd. Tetraethylene glycol dimethyl ether (tetraglyme), ethylene carbonate (EC), and methyl ethyl carbonate (EMC) were purchased from the TCI Chemical. Tetraglyme was distilled under vacuum and dried with activated molecular sieves (4 Å). Lithium hexafluorophosphate (LiPF 6 ), ferrous sulfate (FeSO 4 ), phosphoric acid (H 3 PO 4 ), acetic acid, and hydrogen peroxide (H 2 O 2 ) were purchased from Aladdin. Lithium iron phosphate (LFP) was purchased from Shenzhen Betterui New Materials Group Co., Ltd. Dimethyl sulfoxide-d 6 (DMSO-d 6 ) and 18-crown-6 were purchased from the Shanghai Yuanye Bio-Technology. Argon (N5 grade) and10 % Ar-O 2 (N5 grade) were obtained from Nanjing Special Gas Ltd. Polytetrafluoroethylene emulsion (PTFE) was purchased from Innochem. Celgard separator (25 μm thickness, Celgard), glass fiber separator (GF/F, Whatman), and Super P carbon (Timcal) were purchased from Duoduo Chemical Technology Co. Ltd. Preparation of the composite electrodes The blank carbon electrode, Li 2 CO 3 -carbon composite, and Li 2 CO 3 -Super P-Co 3 O 4 composite (1:1:0.5) electrodes were prepared as described in literature [9] , [28] , [56] . Briefly, a certain amount of Super P, Li 2 CO 3 , and Super P carbon or Li 2 CO 3 , Super P and Co 3 O 4 , and PTFE were mixed and the mixture was ball milled overnight. The mass ratio of active material and binder PTFE is 10:1. A certain amount of well-mixed powder was weighed and absolute ethanol was added to obtain a slurry. The slurry was cast onto pre-washed stainless steel (SS) mesh (100 mesh) and the electrodes were dried under vacuum at 120 °C overnight. The mass loading is 5 mg per electrode. For instance, a Super P- Li 2 CO 3 (1:1) composite electrode contains 2.27 mg Super P, 0.46 mg PTFE, and 2.27 mg Li 2 CO 3 (equivalent to 30.7 μmol). For the 13 C-isotope-labeled electrodes, the Li 2 CO 3 and the Super P were replaced with the Li 2 13 CO 3 and 13 C carbon, respectively. The 13 C-isotope-labeled composite is only obtained by grinding because the 13 C-isotope-labeled substance is too expensive. Preparation of the LFP electrode 80 mg LFP powder, 10 mg Super P, and 100 mg PTFE suspension (10%) were prepared. Firstly, 80 mg LFP and Super P were ground in a mortar to ensure that the LFP and Super P were evenly mixed. 0.1 mL of ethanol was dropped into the mixed powder to wet it and then the PTFE suspension was added to the mixed powder. After LFP-Super P and PTFE were mixed evenly, it was rolled several times with a roller. The final thickness of the electrode is 0.8 mm. The LFP electrode was punched into 12–25 mm diameter and then soaked in a solution (7.2 mL 30% H 2 O 2 and 3 mL acetic acid in 500 mL H 2 O) for 30 min to precharge the LFP. The precharged LFP electrodes were rinsed with water five times to completely remove the residual H 2 O 2 and acetic acid. Finally, the treated LFP electrodes were dried in a vacuum oven overnight and transferred to a glove box for later use. Potential calculation Ag wire was used as a pseudo-reference electrode in a three-electrode cell. We immersed the Ag wire in 1 M LITFSI tetraglyme electrolyte with O 2 to stabilize the potential of the Ag wire. A three-electrode cell with a LFP working electrode was charged and discharged in 1 M LiTFSI-tetraglyme using this Ag wire as the reference electrode. The equilibrium potential of LFP was 0.5 V versus Ag wire. Considering the potential of LFP versus Li + /Li is 3.45 V, the potential of the Ag wire is 2.95 V versus Li + /Li. Therefore, the potentials versus Li + /Li of the experiments in 1 M LiTFSI-tetraglyme could be calculated. All potentials in this manuscript are versus Li + /Li without further notice. DEMS-GC setup A differential electrochemical mass spectrometer (DEMS, Prima BT, Thermo Scientific Ltd.) was coupled with a gas chromatograph (GC, Hope Ltd.) in parallel (Supplementary Fig. 1 ). The GC is equipped with a TCD and an FID detector (including a CO 2 /CO converter). The DEMS cell is based on a customized Swagelok design. It was assembled and charged/discharged in the Ar-filled glove box. The Ar carrier gas carried the evolved gas in the cell into DEMS and GC simultaneously. The typical flow rate of Ag carrier gas is 0.5 mL min −1 and the sweep rate for LSV is 0.05 mV s −1 . The time resolutions of DEMS and GC are 10 seconds and 5 min, respectively. The general gas evolution in chemical reactions was examined by the mass spectrometer (MS, Prima BT) itself. Experiments of Li 2 CO 3 with 1000/5000 ppm H 2 O in 1 M LiTFSI-tetraglyme electrolyte Firstly, 1000 ppm and 5000 ppm H 2 O were added to the 1 M LiTFSI-tetraglyme electrolyte, respectively and the water concentration in the electrolyte was quantified by a Karl Fischer titrator (Mettler Toledo). Then, the gas analysis was conducted in a MS. Generally, 100 mg commercial Li 2 CO 3 was added to a vial that was connected to a MS. After passing in the carrier gas for a while to obtain a steady baseline, 1 mL electrolyte with H 2 O was added to the vial and it was stirred for several hours. The gas evolution was quantified by a MS. Quantification of gas evolution during the charging process The composite electrodes were charged in a homemade differential electrochemical mass spectrometry cell. A piece of precharged LiFePO 4 served as the counter electrode and a piece of silver wire served as the reference electrode. 0.2 mL of 1 M LiTFSI-tetraglyme served as the electrolyte. The water content of the electrolyte was <4 ppm tested by Karl Fischer moisture titrator. To study the impact of the potential on the charging process, the composite electrodes were charged using linear sweep voltammetry (LSV) with a sweep rate of 0.05 mV s −1 . Due to the stability window (4.8 V) of the tetraglyme-based electrolyte, the cell potential was cut off at 4.7 V. Argon was served as the carrier gas and its flow is 0.5 ml/min. The gas evolution was examined by a magnet sector mass spectrometer (Prima BT, Thermo Scientific Ltd.). For the experiments for the chemical route, the Li 2 CO 3 was deliberately separated from the Super P-PTFE composite electrolyte to allow the electrolyte decomposition byproduct to decompose Li 2 CO 3 chemically. Twenty milligrams of commercial Li 2 CO 3 was weighed and dusted to the top of the separator. A piece of Celgard separator (25 μm thickness) was stacked on the Li 2 CO 3 and then a Super P-PTFE composite electrode is stacked on the Celgard. The composite electrode was electronically isolated from Li 2 CO 3 by the Celgard separator. For the 1 M LiTFSI-tetraglyme electrolyte, the cell was charged to 4.7 V and the gas evolution was recorded. For the control experiment with EC/EMC electrolyte, due to the volatile electrolyte, the cell was not purging with Ar carrier gas during the entire charging process. The gas evolution in the headspace was purged with Ar at the end of the charging process to quantify the CO 2 evolution during the entire charging process. A homemade in-line cold trap (−25 °C) was applied to condense the evaporated EMC to minimize the background noise caused by EMC. Quantification of CO The mass-to-charge ( m/z ) ratio of 28 could be contributed by CO, N 2 , and the fragment of CO 2 . To exclude the contribution of the N 2 , the gas inlet of the DEMS was placed inside an Ar-filled glovebox as shown in Supplementary Fig. 1 and the DEMS experiments were conducted inside the glove box at 25 ± 2 °C to minimize the impact of N 2 leakage. The mz = 28 fragment from CO 2 was calibrated with a calibration gas of 1% CO 2 –99% Ar using DEMS. The intensity of the mz = 28 signal is 6.5% of the mz = 44 signal, which is subtracted from the concentration of CO in the calculation. This ratio( mz = 28/ mz = 44) depends on many factors, such as electron voltage, emission current of the filaments, etc. Therefore, this ratio needs to be calibrated for individual MS. A calibration gas of 0.1% CO–99.9% Ar was used for calibration. The CO evolution during the charging process was parallelly quantified by a GC with a TCD and a FID detector (including a CO 2 /CO converter). A FID detector was used to quantify the CO and 1000 ppm CO equals an area of 130 mVs in GC. Thus we could use these results as a reference and qualify the amount of CO in all experiments. Quantification of the solid byproducts The solid Li 2 CO 3 and organic carbon in the composite electrodes were quantified as reported previously [57] . An electrode was placed in a vial that is connected to a MS and 0.5 ml of H 3 PO 4 (2 M) was injected into the vial to react with Li 2 CO 3 to form CO 2 . The CO 2 evolution was quantified by MS. Afterward, Fenton solution (400 μL FeSO 4 + 50 μL of H 2 O 2 (30%)) was added to oxidize the organic carbonates to CO 2 . The released CO 2 was again quantified by a MS. Isotope impurities in Li 2 13 CO 3 and 13 C-carbon A certain amount of Li 2 13 CO 3 reacts with H 3 PO 4 solution in a vial that is connected to a MS. The gas evolution was quantified by MS and shown in Supplementary Fig. 5 . 16.92 μmol of 13 CO 2 and 2.49 μmol 12 CO 2 are identified. Therefore, the ratio between 12 CO 2 and 13 CO 2 is 0.147/1. This result indicates that the commercial Li 2 13 CO 3 sample contains c.a. 15% of 12 C-impurity. The 12 C impurity in the 13 C is determined by a MS as well. The carbon was combusted under a O 2 flow (0.5 mL min −1 ) in a quartz tube that was connected to a MS. The formed 13 CO 2 and 12 CO 2 are quantified and they are 82.42 μmol and 1.27 μmol, respectively. The 13 C sample contains 1.5% of 12 C as an isotope impurity. Identification of 1 O 2 30 mM DMA was added into 1 M LiTFSI-tetraglyme electrolyte as a molecular trap to singlet O 2 . The composite electrode was electrochemical oxidation by linear sweep voltammetry (LSV) with a voltage cutoff of 4.2 V. The electrolyte was extracted from all cell components using DMSO-d 6 for further experiment. 1 H-NMR spectra were recorded on a Bruker Avance III 300 MHz FT NMR spectrometer with autosampler (300.36 MHz, DMSO-d 6 ). We lack an effective way to quantify the 1 O 2 during charging to such a high potential of 4.7 V. On one hand, DMA decomposes above 4.2 V and thus we cannot use DMA to detect 1 O 2 at 4.7 V. However, there is only a small portion (<5%) of Li 2 CO 3 decomposes below 4.2 V and the amount of 1 O 2 at this stage is low, which could not represent the overall reaction up to 4.7 V. For the aspect of energy, more 1 O 2 would form at a higher potential. On the other hand, the NMR is only a semi-quantitative technique. Thus probing DMA-O 2 using NMR could only confirm the formation of 1 O 2 but it could not provide a reliable quantification of such a low amount of 1 O 2 . The NMR of the electrolyte in a cell with Co 3 O 4 is shown in Supplementary Fig. 18 . The cell was charged by LSV to 4.2 V. The electrolyte was extracted from all cell components using DMSO-d 6 . The signals of DMAO 2 in both samples are too weak to compare quantitatively. Chemical experiments between reactive oxygen species and carbon The purpose of this ex situ chemical experiment is to identify the products of reactive oxygen species attacking 13 C-carbon. We try to prove the feasibility that 1 O 2 attacks 13 C-carbon to form 13 CO 2 and 13 CO, which is detected during the charging process of the cell with Li 2 CO 3 . Meanwhile, our results show that superoxide species could not oxidize 13 C-carbon to form 13 CO 2 and 13 CO. Singlet oxygen was obtained by the disproportionation of superoxide species, which is KO 2 and Li + here. Briefly, a varying amount of 13 C-carbon and 22 mg KO 2 powder was added to a vial that is connected to a MS before the solution is added into the vial. The carrier gas will be passed for a period to eliminate the residual gas in the vial. Then, 1 mL high concentration lithium salt electrolyte (4 M LiTFSI here) was injected into the vial to react with KO 2 to disproportionate to produce 1 O 2 . 1 O 2 immediately oxidized 13 C-carbon to evolve 13 CO 2 and 13 CO. The produced gases were detected by a MS. An excess amount of KO 2 was used here to produce a large amount of 1 O 2 . So far, we could not quantify the amount of 1 O 2 produced in this disproportionation reaction of KO 2 and Li + . Here, the experiments were carried out without applying a potential, namely at “OCV”. The reactivity of carbon and the ratio of CO 2 /CO may change when voltage is applied. The impact of potential in the side-reaction of 1 O 2 and 13 C is not the focus of this work. Also, when a high potential is applied to the carbon substrate, electrode decomposition will take place, which makes the situation complicated to decouple these factors. Here, we mainly focus on Li 2 CO 3 electro-oxidation. Although carbon oxidation accompanies Li 2 CO 3 decomposition, it only contributes to ~10% of the total CO 2 evolution. A control experiment of superoxide attacking 13 C-carbon was carried out to make a comparison. Superoxide was obtained as previously reported [52] . In brief, firstly, argon was used to exclude the dissolved gas such as oxygen in the tetraglyme solvent. Then, 71 mg KO 2 and 264 mg 18-crown-6 were added to 10 mL tetraglyme electrolyte and stirred for four hours to maximize the concentration of the O 2 − (sol) . The electrolyte was centrifuged and the supernatant also was injected with argon to get out the dissolved oxygen produced by the KO 2 attack electrolyte for further experiment. Finally, varying amounts of 13 C-carbon powder were added to a vial and 1 mL supernatant was injected into the vial for the source of superoxide. The produced gases were detected by a MS. In the charging process of the cell, because Li 2 CO 3 has ultralow ionic and electronic conductivities, its decomposition takes place at the 13 C|Li 2 CO 3 solid-solid interface (namely the contact points between 13 C particles and Li 2 CO 3 particles). Therefore, the decomposition product, 1 O 2 , is just formed at this interface, which is very close to 13 C, and thus it is easy to attack 13 C. Therefore, the ratio between 1 O 2 and 13 C is high. On the contrary, in the chemical experiments described above, 1 O 2 originates from the disproportionation of superoxide in the solution phase. Although 13 C was added to the solution and stirring was applied, the fresh 1 O 2 forms from the disproportionation process in the electrolyte and it first attacks the electrolyte. Only a small portion of 1 O 2 would diffuse to the surface of the suspended 13 C in the electrolyte and react with 13 C. In addition, the ratio of releasing 1 O 2 from disproportionation is still unknown, which is highly likely below 10%. Freunberger et al show that more 1 O 2 forms during the charging process than in the discharging process involving disproportionation. Quenching 1 O 2 Once the 1 O 2 forms in the electrolyte, it is too late to stabilize it and it rapidly attacks the electrolyte and carbon substrate. Therefore, our strategy is to stabilize this intermediate/precursor which further produces singlet oxygen, rather than to quench the 1 O 2 after its formation in the electrolyte. In this case, we hope that Co 3 O 4 binds the intermediate (namely the precursor of 1 O 2 , e.g. CO 4 2− ) into a complex such as Co 3 O 4 -CO 4 , before 1 O 2 is formed and dissolved in the electrolyte. Our experimental results show that Co 3 O 4 makes some positive effects, but it is not good enough. If it works properly, the ratio(CO 2 /O 2 ) should be 2 according to the equ 1a, but the ratio(CO 2 /O 2 ) Co3O4 is 6.7, much higher than 2. It might be a feasible strategy to inhibit 1 O 2 formation but there are still lots of work that need to be done.